Isotopic constraints on biogeochemical cycling of copper in the ocean Trace elements and their isotopes are being actively studied as powerful tracers in the modern ocean and as proxies for the palaeocean. Although distributions and fractionations have been reported for stable isotopes of dissolved Fe, Cu, Zn and Cd in the ocean, the data remain limited and only preliminary explanations have been given. Copper is of great interest because it is either essential or toxic to organisms and because its distribution reflects both biological recycling and scavenging. Here we present new isotopic composition data for dissolved Cu (δ 65 Cu) in seawater and rainwater. The Cu isotopic composition in surface seawater can be explained by the mixing of rain, river and deep seawater. In deep seawater, δ 65 Cu becomes heavier with oceanic circulation because of preferential scavenging of the lighter isotope ( 63 Cu). In addition, we constrain the marine biogeochemical cycling of Cu using a new box model based on Cu concentrations and δ 65 Cu. Copper plays an important role as a micronutrient for organisms in the ocean, but high concentrations of the free Cu 2+ ion are toxic [1] . Dissolved Cu has concentrations of 0.5–6 nmol kg −1 in seawater and mostly complexes with organic ligands, which results in very low concentrations (fmol kg −1 to pmol kg −1 ) of the free Cu 2+ ion [2] . Vertical distributions of dissolved Cu are of the nutrient-scavenging hybrid type [3] . Generally, the concentrations of nutrient-type trace metals (for example, Zn, Ni and Cd) are low in the surface layer of the ocean because of biological uptake. However, the concentrations increase with depth, showing a mid-depth maximum because of remineralization from settling particles. By contrast, the concentration of dissolved Cu gradually increases with depth to the bottom. Such distributions have been interpreted to be caused by a combination of scavenging throughout the water column and a supply from the uppermost layer of benthic sediments, where scavenged Cu is recycled to overlying seawater via early diagenesis [4] , [5] . Copper has two stable isotopes, 63 Cu and 65 Cu, and its isotopic composition is reported as δ 65 Cu(‰)=[( 65 Cu/ 63 Cu) sample /( 65 Cu/ 63 Cu) NIST SRM 976 −1] × 10 3 . To date, only a few vertical profiles of dissolved δ 65 Cu in the ocean have been reported [6] , [7] , [8] , [9] . The reported δ 65 Cu values (0.44–1.44‰) were substantially heavier than typical values for the solid Earth (~0‰) [10] , [11] . However, as there are relatively large uncertainties in the reported data, it has been difficult to elucidate intra-ocean distributions. This is partly due to analytical difficulties in the determination of δ 65 Cu caused by the interference of matrices and the inapplicability of the so-called double-spike technique. Recently, we developed a simple and precise analytical method for δ 65 Cu based on a chelating resin extraction technique [12] . Here we use this method to present new isotopic data of compositions of dissolved Cu (δ 65 Cu) in seawater from the North and South Atlantic, South Indian and North Pacific oceans. We also present new data from rainwater samples collected from urban and rural regions. Using these data, the Cu isotopic composition in surface seawater is explained in an oceanographic context. In deep seawater, δ 65 Cu values show a linear correlation with apparent oxygen utilization (AOU), which suggests δ 65 Cu becomes heavier with oceanic circulation because of preferential scavenging of the lighter isotope ( 63 Cu). Our data show that the stable isotopic values of trace metals may change systematically with the age of deep water. In addition, we propose a new box model for Cu in the ocean based on the combination of Cu concentration and δ 65 Cu, constraining the marine biological cycling of Cu. Seawater analyses The observed oceanic stations are shown in Fig. 1 . 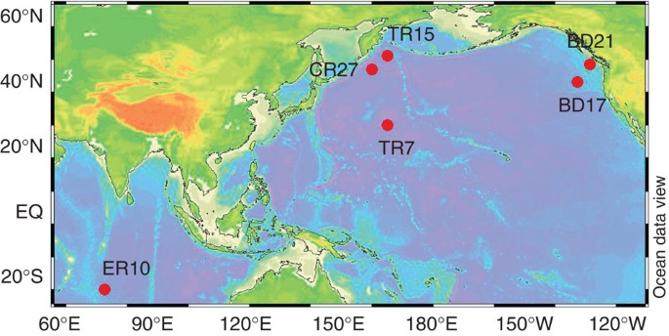Figure 1: Station locations. Samples for the analysis of δ65Cu were collected at these stations during R/VHakuho-marucruises. The numbers of samples are 10 at TR7, 10 at TR15, 10 at CR27, 14 at BD17, 12 at BD21 and 18 at ER10. This figure was produced using Ocean Data View13. All seawater data are summarized in Supplementary Table 1 . The vertical profiles of dissolved Cu concentration and δ 65 Cu for each station are presented in Supplementary Fig. 1 , and representative profiles are shown in Fig. 2 . The Cu concentrations were in the range of 0.6–4.6 nmol kg −1 , and the profile at station ER10 agreed well with that determined in separate samples collected at the same station in our previous research ( Supplementary Fig. 2 ) [14] . The δ 65 Cu values ranged from +0.41‰ to +0.85‰, which was lighter than values determined by a Mg(OH) 2 co-precipitation technique (+0.50 to 1.44‰) [7] , [8] at other stations and similar to values determined by a solvent extraction technique (+0.44 to 0.78‰) [6] , [9] at other stations ( Supplementary Fig. 3 ). The vertical samples from the GEOTRACES Atlantic intercalibration station (Bermuda Atlantic Time-series Study, BATS) have been analysed using a solvent extraction technique by Thompson et al. [9] The reported δ 65 Cu value (0.56±0.09‰) for a 2,000-m depth sample was higher than our value (0.41±0.05‰). Unfortunately, we are not able to investigate the causes because the BATS samples have been exhausted. Recently, we performed an intercalibration of δ 65 Cu with a group from ETH, Zurich (see Acknowledgements section for details), using seawater collected at a station near the Japan Trench, of which details are described in the Supplementary Methods . The ETH group used a new method based on Al(OH) 3 co-precipitation [15] , which gave results consistent with ours ( Supplementary Fig. 4 ). Figure 1: Station locations. Samples for the analysis of δ 65 Cu were collected at these stations during R/V Hakuho-maru cruises. The numbers of samples are 10 at TR7, 10 at TR15, 10 at CR27, 14 at BD17, 12 at BD21 and 18 at ER10. This figure was produced using Ocean Data View [13] . 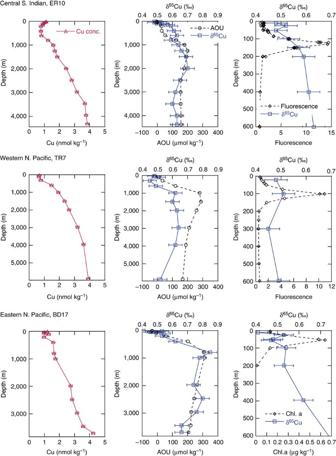Figure 2: Representative vertical profiles of the concentration and isotopic composition of Cu. Magenta triangles indicate Cu concentration. Blue squares and black circles indicate δ65Cu and apparent oxygen utilization (AOU), respectively. Black diamonds indicate fluorescence or chlorophyll a (Chl. a). The error bars are 2 s.d. of ±0.045‰ for δ65Cu and ±0.11 nmol kg−1for Cu concentration, as described in the Methods section. The vertical profiles at all stations are shown inSupplementary Fig. 1. Full size image Figure 2: Representative vertical profiles of the concentration and isotopic composition of Cu. Magenta triangles indicate Cu concentration. Blue squares and black circles indicate δ 65 Cu and apparent oxygen utilization (AOU), respectively. Black diamonds indicate fluorescence or chlorophyll a (Chl. a). The error bars are 2 s.d. of ±0.045‰ for δ 65 Cu and ±0.11 nmol kg −1 for Cu concentration, as described in the Methods section. The vertical profiles at all stations are shown in Supplementary Fig. 1 . Full size image The vertical profiles of δ 65 Cu in this work showed a common feature: δ 65 Cu was ~0.5‰ in the surface layer and became heavier at depth. Station BD21 above the Juan de Fuca Ridge had a minimum Cu concentration at a depth of 2,300 m, reflecting the effect of a hydrothermal plume [16] . There were, however, no significant variations in δ 65 Cu. Rainwater analyses We also determined δ 65 Cu in rainwater for the first time ( Table 1 ). Rainwater was sampled from rural and urban regions in Japan. The dissolved δ 65 Cu values were in the narrow range of −0.12 to +0.03‰ and did not show significant differences depending on location and time, whereas the Cu concentrations varied largely (1.1–23.5 nmol kg −1 ), which may reflect various contributions of anthropogenic input. It has been reported that δ 65 Cu values were ~0‰ for leachable fractions of marine aerosols [11] and bulk loess [17] . Rainwater would scavenge both atmospheric dusts and anthropogenic aerosols during precipitation. Therefore, it seems reasonable to presume the δ 65 Cu value for atmospheric input to be zero. Table 1 Rainwater analysis results. Full size table Copper isotopes in surface seawater In Fig. 3 , the δ 65 Cu in surface seawater is plotted against the reciprocal Cu concentration together with the ranges and averages of deep seawater, rural rainwater and river water [8] . Assuming that average surface seawater is a mixture of average rural rainwater, average river water and average deep seawater, the plot would be located in the magenta triangle. Evaporation that is another important factor to control salinity; it would increase the Cu concentration but not change the δ 65 Cu. However, the surface water data are shifted to the right of the triangle, indicating there must be other processes that decrease the dissolved Cu concentration (up to one tenths) while keeping the δ 65 Cu values constant. The most likely process is phytoplankton uptake and adsorption of Cu onto the phytoplankton surface. It is well known that these processes produce biogenic sinking particles in the surface layer and they transport trace metals to the deep layer. Our data suggest that uptake and adsorption by phytoplankton in the open ocean does not cause significant fractionation of Cu isotopes. To clarify mechanisms controlling the Cu concentration and δ 65 Cu, it is informative to compare Cu and Cd in the ocean. For vertical profiles of dissolved Cd, the isotopic ratio (ε 114 Cd) correspondingly increases with a decrease in the concentration in the surface layer and decreases with an increase in the concentration from the surface to the intermediate layer, because biological uptake causes isotopic fractionation of Cd [18] , [19] , [20] . Therefore, the profile of ε 114 Cd from the surface to the intermediate layer becomes a mirror image of the concentration, and ε 114 Cd linearly correlates with the logarithm concentration in the surface layer because of Rayleigh fractionation during biological uptake [18] , [19] , [20] , [21] . However, δ 65 Cu does not change correspondingly to the Cu concentration from the surface to the intermediate layer ( Fig. 2 and Supplementary Fig. 1 ), and does not correlate with the logarithmic concentration in the surface layer ( Supplementary Fig. 5 ). These facts also indicate biological processes cause insignificant fractionation of the Cu isotopes. 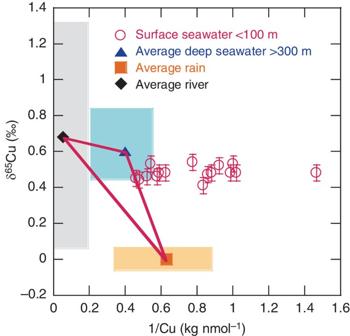Figure 3: δ65Cu vs reciprocal Cu concentration for surface seawater (<100 m). The error bars of the magenta circles are 2 s.d. of ±0.045‰. The blue, black and orange shaded areas indicate the ranges of the data for deep seawater, river water and rural rain, respectively. The magenta triangle indicates the possible range of mixtures of average deep seawater, river water and rainwater. The surface water data shifted to the right of the triangle indicate that other processes decrease the dissolved Cu concentration in the surface seawater. Figure 3: δ 65 Cu vs reciprocal Cu concentration for surface seawater (<100 m). The error bars of the magenta circles are 2 s.d. of ±0.045‰. The blue, black and orange shaded areas indicate the ranges of the data for deep seawater, river water and rural rain, respectively. The magenta triangle indicates the possible range of mixtures of average deep seawater, river water and rainwater. The surface water data shifted to the right of the triangle indicate that other processes decrease the dissolved Cu concentration in the surface seawater. Full size image Copper isotopes in deep seawater Given that uptake and adsorption of Cu by phytoplankton does not cause fractionation of Cu isotopes, biogenic sinking particles would have the same δ 65 Cu value as surface seawater. Copper regenerated through decomposition of the biogenic sinking particles should produce δ 65 Cu values in deep seawater, which are the same as those in surface seawater under this assumption. However, observed δ 65 Cu in deep seawater is heavier than that in surface seawater. In addition, the profiles of δ 65 Cu are similar to those of AOU ( Fig. 2 and Supplementary Fig. 1 ). All δ 65 Cu values are plotted against AOU, revealing a positive correlation ( R 2 =0.60, n =77; Fig. 4a ). In the layer deeper than 2,000 m, δ 65 Cu vs AOU shows a stronger correlation ( R 2 =0.70, n =25; Fig. 4b ). Because AOU is a measure of the age of deep water, these data imply that δ 65 Cu increases through deep water circulation. When the Cu concentration is plotted against AOU, there is also a weak correlation ( R 2 =0.31, n =77, Fig. 5 ). 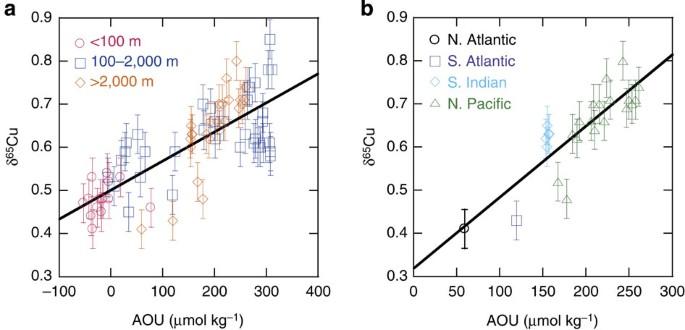Figure 4: δ65Cu vs AOU for seawater. The error bars for δ65Cu are 2 s.d. of ±0.045‰. (a) All δ65Cu values were plotted against apparent oxygen utilization (AOU). The solid line was determined by a regression analysis of all plots: δ65Cu=0.00067 × AOU+0.50,R2=0.60,n=77,P<0.001. (b) δ65Cu values were plotted against AOU in deep seawater (>2,000 m). The solid line was determined by a regression analysis of all plots: δ65Cu=0.0016 × AOU+0.32,R2=0.70,n=25,P<0.001. Figure 4: δ 65 Cu vs AOU for seawater. The error bars for δ 65 Cu are 2 s.d. of ±0.045‰. ( a ) All δ 65 Cu values were plotted against apparent oxygen utilization (AOU). The solid line was determined by a regression analysis of all plots: δ 65 Cu=0.00067 × AOU+0.50, R 2 =0.60, n =77, P <0.001. ( b ) δ 65 Cu values were plotted against AOU in deep seawater (>2,000 m). The solid line was determined by a regression analysis of all plots: δ 65 Cu=0.0016 × AOU+0.32, R 2 =0.70, n =25, P <0.001. 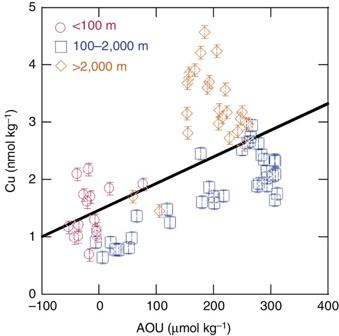Figure 5: Cu concentration vs AOU in the ocean. The error bars are 2 s.d. of ±0.11 nmol kg−1. The solid line was defined as: [Cu]=0.0046 × AOU+1.5,R2=0.31,n=77,P<0.001. Full size image Figure 5: Cu concentration vs AOU in the ocean. The error bars are 2 s.d. of ±0.11 nmol kg −1 . The solid line was defined as: [Cu]=0.0046 × AOU+1.5, R 2 =0.31, n =77, P <0.001. Full size image In the case of Cd, the dissolved concentration is very low (~0.001 nmol kg −1 ) in the surface layer because of biological uptake, and it is high in the deep layer (~1 nmol kg −1 ) because of remineralization from biogenic particles; it also increases along the global deep circulation [3] . Because there is a significant correlation between Cd and phosphate, the distribution of Cd is dominated by biogeochemical recycling. The isotopic composition of Cd is heavier in surface seawater (ε 114/110 Cd=10–40 with respect to the JMC Cd Münster solution) than in deep seawater (ε 114/110 Cd=~3) that is almost uniform in the world ocean [18] , [19] , [20] . Biological uptake depletes the Cd concentration and preferentially leaves isotopically heavy Cd in surface seawater. It is suggested that Cd in a replenished surface seawater reservoir is originally characterized by ε 114/110 Cd=~3 and that this Cd is almost quantitatively transported by biogenic sinking particles from the surface to depth and remineralized in deep water; thus, the Cd isotopic composition of deep water is homogeneous, whereas the Cd concentration increases along with deep water circulation. The δ 65 Cu in deep seawater appears to be controlled by a ubiquitous effect throughout the water column and deep water pathway because δ 65 Cu correlates with AOU. Copper is more strongly scavenged than other recycled-type trace metals such as Cd [3] , [5] . The scavenging is likely the reason that δ 65 Cu is heavy in the deep layer and becomes heavier with the age of deep seawater. If this is true, 63 Cu would be preferentially adsorbed to sinking particles and preserved in sinks. The low linearity of Cu concentration against AOU ( Fig. 5 ) would be due to the combination of scavenging throughout the water column and supply from sediments through decomposition of the organic fraction of sinking particles. The Cu released from sediments most likely has a δ 65 Cu value similar to that in seawater near the bottom, resulting in the linearity of δ 65 Cu vs AOU. Box model for Cu in the modern ocean We present a new box model for Cu based on both concentration and isotopic composition ( Fig. 6 and Supplementary Table 2 ). This model assumes a steady state for the modern ocean. In this model, the global ocean is divided simply into a euphotic layer and a deep layer at a depth of 100 m. A thin layer on the sediment surface is considered as the box of the ‘scavenged layer’, where organic matter is decomposed during early diagenesis [22] . In Fig. 6 , the black figures are observed or previously published values, as described below. 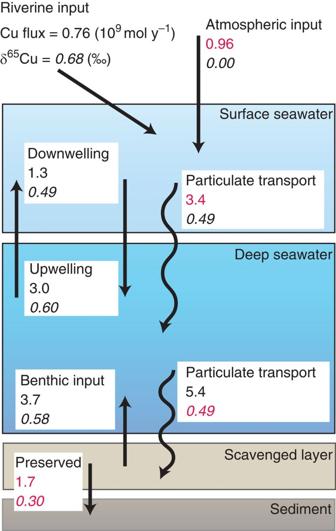Figure 6: Box model for Cu cycling in the ocean based on both elemental concentration and isotopic ratio. The Roman and italic values below the process names represent Cu flux in units of 109mol yr−1and δ65Cu values in ‰, respectively. Black figures indicate observed values and magenta figures indicate values calculated based on mass balance. Magenta figures are values calculated using the following equations [11] , which assumes a steady state for each box: Figure 6: Box model for Cu cycling in the ocean based on both elemental concentration and isotopic ratio. The Roman and italic values below the process names represent Cu flux in units of 10 9 mol yr −1 and δ 65 Cu values in ‰, respectively. Black figures indicate observed values and magenta figures indicate values calculated based on mass balance. Full size image where F in and F out represent an input and output flux for the box, and δ in and δ out represent δ 65 Cu values of F in and F out , respectively. Based on this work, the depth-weighted averages of Cu concentration and δ 65 Cu are 1.1 nmol kg −1 and 0.49‰ in surface seawater and 2.5 nmol kg −1 and 0.60‰ in deep seawater, respectively. The water mixing rate between the upper box and lower box is assumed to be 1.2 × 10 15 m 3 yr −1 , which has been determined from 14 C data [23] . We assumed that the main inputs of dissolved Cu to the ocean are riverine and atmospheric inputs. The reported riverine input of dissolved Cu to the ocean among four studies [4] , [8] , [24] , [25] was in the range of 6−9 × 10 8 mol yr −1 , and the average value of 7.6 × 10 8 mol yr −1 was applied to our model. The removal rate of dissolved Cu from the ocean was estimated to be ~4.0 nmol kg −1 yr −1 by using a vertical advection diffusion model [4] , [5] . By multiplying this value by the total ocean volume (1.35 × 10 21 kg), the scavenging flux of Cu in the ocean was estimated to be 5.4 × 10 9 mol yr −1 . Riverine input δ 65 Cu was determined in rivers worldwide; the rivers account for approximately one-quarter of all riverine discharge to the ocean [8] . The discharge-weighted average of 0.68‰ of these rivers was used in our model. The δ 65 Cu of atmospheric input was assumed to be 0‰ because δ 65 Cu values are ~0‰ for rainwater, leachable fractions of marine aerosols [11] and loess [17] . It was assumed that the δ 65 Cu of sinking particles (of mainly biogenic origin) from surface water was the same as the δ 65 Cu of ambient surface seawater (that is, 0.49‰), because isotopic fractionation during phytoplankton uptake and adsorption onto phytoplankton surface is expected to be insignificant, as described above. The δ 65 Cu of the benthic flux from the scavenged layer to deep seawater was assumed to be the global average of 0.58‰. This value is the average of δ 65 Cu in seawater samples nearest the bottom of the ocean. The unknown Cu fluxes that were calculated by this model are those of supply from the atmosphere, transport by sinking particles from the surface, preservation in sediments and return from the scavenged layer to deep water. The unknown δ 65 Cu values calculated by this model are those of the transporting flux by sinking particles in deep water and the preserved flux into sediments. From our data we infer that the δ 65 Cu values in surface seawater are mainly controlled by supply from rivers, the atmosphere and deep seawater. Biological uptake does not appear to cause significant isotopic fractionation of Cu in the open ocean. δ 65 Cu values in deep seawater are heavier than those in surface seawater and become heavier with the age of deep seawater, likely due to preferential scavenging of the light isotope ( 63 Cu). Biological fractionation of Cu isotopes has not yet been sufficiently elucidated in the literature. There are only a few studies concerning isotopic fractionation of Cu by phytoplankton. Laboratory experiments have shown that uptake by several diatoms caused no significant fractionation or slight enrichment of the heavy Cu isotope ( 65 Cu) when the initial Cu concentration was ~200 nmol l −1 (ref. 26 ). However, a geochemical study in the Garonne River suggested that diatom species prefer the light Cu isotope ( 63 Cu) [27] . Thus, it is necessary to determine the δ 65 Cu of natural phytoplankton in the open ocean in future work. We suggest that Fe-Mn oxides may be a major sink of Cu in the oxic ocean. δ 65 Cu values of Fe-Mn nodules are 0.33±0.23‰ (average±2 s.d., n =14) in the Pacific, 0.25±0.26‰ ( n =8) in the Atlantic and 0.31±0.23‰ ( n =31) in the world’s oceans collectively [10] ; the δ 65 Cu values of Fe-Mn crusts are 0.54±0.07‰ ( n =8) in the Pacific, 0.33±0.15‰ ( n =8) in the Atlantic and 0.44±0.23‰ ( n =16) in major ocean basins collectively [11] . Thus, δ 65 Cu of Fe-Mn crusts and nodules is lighter than that of dissolved Cu in the ocean. Furthermore, the δ 65 Cu of Fe-Mn crusts is significantly heavier in the Pacific than in the Atlantic ( P =0.01). These data are consistent with preferential scavenging of 63 Cu and gradual accumulation of 65 Cu in seawater via global ocean circulation. This view, however, seems contrary to experimental results on adsorption of Cu isotopes on Fe oxyhydroxides [26] , [28] , which indicate enrichment of the heavy Cu isotope onto oxide surfaces in NaNO 3 solutions or mixtures of acidic drainage and river water. The discrepancy may be caused by differences in conditions, such as pH, Cu concentration and organic ligand concentration, between experimental solutions and natural seawater. In addition, it has been reported that Cu is associated with Mn and not Fe in Fe-Mn crusts [29] . Isotopic fractionation between free Cu and organic ligand-bound Cu could also be important for Cu isotopes in seawater, because Cu is mostly complexed with organic ligands. In a laboratory experiment, humic acid preferentially formed complexes with the heavy Cu isotope [30] . It is therefore likely that the complexation of Cu with dissolved organic ligands in seawater also causes mass fractionation of Cu, because the organic ligands and humic acid most likely have the same functional groups. Furthermore, Cu is contained not only in the Fe-Mn oxide fraction but also in the organic fraction of sinking particles [31] , [32] . Thus, understanding isotopic fractionation during scavenging of dissolved Cu from seawater is not straightforward. It was originally proposed in a previous field study of rivers and oceans that there is equilibrium partitioning of isotopes between heavy Cu bound to organic ligands in the dissolved phase and light Cu adsorbed to particles [8] . This hypothesis is consistent with our explanation of light Cu scavenging. In the box model using both the Cu concentration and δ 65 Cu ( Fig. 6 ), we constrained the transporting flux of Cu from surface to deep water by sinking particles to be 3.4 × 10 9 mol yr −1 . The residence time for dissolved Cu in surface water (<100 m) is ~9 years, which is consistent with previous estimates of 3.2–11.7 years [5] , [33] . The calculated preservation flux of Cu into sediments is 1.7 × 10 8 mol yr −1 . The overall residence time of Cu in the ocean is calculated by dividing the average concentration by the preservation flux. Our estimate of the overall residence time of Cu is 2,000 years, which is within the range of literature values (1,700–6,400 years) [4] , [11] . The calculated δ 65 Cu of preserved Cu in sediments is +0.30‰, which is quite similar to the averages reported for Fe-Mn oxides [10] , [11] . We constrained the atmospheric input of dissolved Cu to be 9.6 × 10 8 mol yr −1 . Our model suggests that the present atmospheric input of Cu is comparable to the riverine input. A significant correlation was found between Cu and 210 Pb in surface seawater, implying a strong atmospheric supply of Cu, as 210 Pb is a tracer for atmospheric input [4] . Boyle et al. [4] estimated both the atmospheric and riverine Cu input to be 6.0 × 10 8 mol yr −1 , which is similar to our results. However, our value is significantly larger than the natural atmospheric input previously estimated at 5.4 × 10 7 mol yr −1 , which was obtained by multiplying the total dust flux by the mean crustal Cu concentration and solubility [11] . Two possible explanations are given to rationalize this difference. First, it is possible that the Cu concentration and solubility in marine aerosols would be different from those in the continental crust. The enrichment factor of Cu relative to Al in marine aerosols varies over a large range of 1–200 compared with the continental crust [25] . The solubility of Cu in aerosols has a wide range of 15–86% (ref. 34 ). It has been suggested that the enriched and soluble Cu in aerosols are from anthropogenic sources [34] , [35] , [36] . However, Maring et al. evaluated the source of Cu enrichment in aerosols near Enewetak in the North Pacific, suggesting that atmospheric soluble Cu is from primary natural origins and that soil organic matter enriched in Cu could be a significant source of soluble Cu [37] . If anthropogenic Cu has significantly affected atmospheric input as we estimate, then the steady-state assumption is imperfect for the modern ocean, because anthropogenic inputs would have substantially increased in the recent ~100 years, whereas the overall oceanic residence time of Cu is thousands of years. Second, other fluxes to the open ocean surface may have an effect. One possible flux is from the continental shelf sediment, where a portion of Cu is derived from the reduction of primary terrigenous metal oxides [38] . The δ 65 Cu value of this flux would also be close to the crustal value (0‰) and lighter than that of surface seawater. If these fluxes are included in our box model, then our estimate of atmospheric input may decrease. As described above, some uncertainties remain in our box model. Our results, however, confirm possibilities of this new box model based on both concentration and isotopic composition of trace metals. Seawater samples The South Indian and North Pacific seawater samples were collected during the R/V Hakuho-maru cruises KH 09-4, KH 10-2, KH 11-7 and KH 12-4 using a clean sampling system [14] . In a clean booth, seawater was filtered through a 0.2-μm cartridge filter (Acro pak, Pall), acidified with HCl to pH 1.7–2.2, and stored in 2-l or 4-l LDPE bottles (Nalgene bottle, Thermo Fisher Scientific) or 6-l LDPE cubic bags (Lontainer, Sekisui Seikei), which were pre-cleaned by overnight treatment with 4 M HCl followed by rinsing with deionized water. The North Atlantic sample was a GEOTRACES reference material collected at BATS during the US-GEOTRACES KN193-5 cruise of the R/V Knorr . The South Atlantic sample was collected at Station 3 during the UK-GEOTRACES D357 cruise of the RSS Discovery . Rainwater samples Rainwater was collected from two sites using pre-cleaned polyethylene funnels and cubic bags (Lontainer) or 2-l LDPE bottles. One site was on the roof of the main building of the Institute for Chemical Research, which is located in an urban area of Honshu Island, Japan. The other site was on top of Mt. Kajigamori, which is located in a rural area of Shikoku Island. Rainwater samples were filtered through a 0.22-μm filter (Millipore) and acidified with HCl to pH 1.7–2.1. Analytical procedure of δ 65 Cu and Cu Copper concentration and isotopic composition were determined as described in a previous paper [12] . Briefly, Cu in seawater or rainwater was collected using a column of Nobias chelate PA-1 resin (Hitachi High Technologies) followed by elution with 1 M HNO 3 . The eluate was evaporated to dryness, and the residue was re-dissolved with 10 M HCl. The sample was passed through a column of anion exchange resin (AG MP-1, Bio-Rad); additional 10 M HCl was then passed through the column to remove co-existing elements, followed by the elution of Cu with 5 M HCl. This eluate was evaporated to dryness and the residue was re-dissolved with 1 M HNO 3 . Finally, the 1 M HNO 3 solution was re-evaporated and the residue was re-dissolved with 0.4 M HNO 3 , yielding the pre-concentrated sample. One hundred micrograms of the pre-concentrated sample was diluted with 0.4 M HNO 3 by a factor of ~10 and used for measurement of Cu concentration. Co-existing Na, Mg, Ba, Ni, Zn, Cr and Ti were also measured to ascertain whether these interfering elements possessed concentrations sufficiently low to permit accurate Cu isotopic measurements. When the Na (p.p.b. )/Cu (p.p.b.) ratio in the pre-concentrated sample was higher than 1, the solution was not used for discussion. For the Cu isotopic measurement, which used a multicollector ICP-MS (Thermo Finnigan Neptune or Neptune Plus, Thermo Fisher Scientific), the final solution was diluted to adjust the Cu concentration to 50 p.p.b. and Zn was added to give a solution of 100 p.p.b. for external normalization. The precision of this method was evaluated previously by repeated analyses of coastal seawater to be ±0.07‰ (±2 s.d., n =6) [12] . In this study, 34 samples were each divided into two aliquots and analysed in duplicate, resulting in an average 2 s.d. of 0.045‰ ( n =34) for δ 65 Cu and 0.11 nmol kg −1 ( n =34) for Cu concentration. These values are shown as error bars in the figures. How to cite this article: Takano, S. et al. Isotopic constraints on biogeochemical cycling of copper in the ocean. Nat. Commun. 5:5663 doi: 10.1038/ncomms6663 (2014).